interleukin-11induces and maintains progenitors of different cell lineages duringXenopustadpole tail regeneration Unlike mammals, Xenopus laevis tadpoles possess high ability to regenerate their lost organs. In amphibians, the main source of regenerated tissues is lineage-restricted tissue stem cells, but the mechanisms underlying induction, maintenance and differentiation of these stem/progenitor cells in the regenerating organs are poorly understood. We previously reported that interleukin-11 ( il-11 ) is highly expressed in the proliferating cells of regenerating Xenopus tadpole tails. Here, we show that il-11 knockdown (KD) shortens the regenerated tail length, and the phenotype is rescued by forced- il-11 -expression in the KD tadpoles. Moreover, marker genes for undifferentiated notochord, muscle, and sensory neurons are downregulated in the KD tadpoles, and the forced- il-11 -expression in intact tadpole tails induces expression of these marker genes. Our findings demonstrate that il-11 is necessary for organ regeneration, and suggest that IL-11 plays a key role in the induction and maintenance of undifferentiated progenitors across cell lineages during Xenopus tail regeneration. Some lower vertebrates, such as fish and amphibians, have a prominent ability to regenerate their lost organs compared to mammals [1] . Xenopus laevis tadpoles can regenerate their lost tails, including all tissues that comprise tails, such as the notochord, muscle, spinal cord and other tissues, after amputation, and are used as model animals for the study of vertebrate organ regeneration. In the regeneration of X. laevis tails [2] or axolotl limbs [3] , the main sources of the regenerated organs are lineage-restricted tissue stem cells. Although the mechanisms underlying the synergistic induction, maintenance, and differentiation of these stem and/or progenitor blastema cells during organ regeneration are fundamental in organ regeneration, the detailed molecular mechanisms are not well understood. We previously reported that interleukin-11 ( il-11 ) is highly expressed in the proliferating cells in regenerating X. laevis tadpole tails [4] , raising the possibility that IL-11 plays a crucial role in Xenopus tadpole tail regeneration. IL-11 is a member of IL-6 family, and its signalling cascade has been extensively studied in mammals [5] . IL-11 binds to both IL-11 receptor alpha (IL11RA) and IL-6 signal transducer (IL6ST, also known as GP130) [6] , [7] , and transduces signals through IL6ST [8] . IL6ST is a receptor subunit common to all IL-6 family cytokines. Activated IL6ST phosphorylates signal transducer and activator of transcription (Stat) 1 and 3 [9] , and phosphorylated Stat1 and Stat3 translocate to the nucleus to activate the transcription of target genes [10] , [11] . IL-11 also activates the mitogen-activated protein/extracellular signal-regulated kinase kinase (MEK) pathway [12] , and the phosphatidylinositol-3 kinase (PI3K) pathway [13] . Some members of the IL-6 family are involved in regulating the differentiation of stem/progenitor cells. For example, IL-6 treatment differentiates B lymphocytes to antibody-forming cells [14] . Leukaemia inhibitory factor (Lif) inhibits the differentiation of mouse embryonic stem cells [15] , [16] . IL-11 treatment is reported to maintain the expression of undifferentiated markers in human embryonic stem cells [17] . il-11 is also suggested to be involved in regeneration. il-11 is reported to be expressed in the regenerating heart of zebrafish, and forced expression of a dominant negative form of Stat3 inhibits the proliferation of cardiomyocytes and heart regeneration [18] . Based on these findings, Fang et al. speculated that IL-11 is a candidate upstream molecule of the Stat3 pathway that is responsible for the proliferation of cardiomyocytes during regeneration. The precise role of il-11 in regeneration of organs comprised of various tissues, however, is not clear. Here, we produced il-11 knockeddown (KD) tadpoles using the CRISPR/Cas9 system to show that il-11 is necessary for tail regeneration in X. laevis tadpoles. In addition, the shortened regenerated tails, a phenotype of the il-11 KD tadpoles, is rescued by forced expression of il-11 at the amputated tail stumps. In the amputated tail stumps of the il-11 KD tadpoles, marker genes for undifferentiated notochord, muscle and sensory neurons are downregulated compared to control tadpoles. Furthermore, forced expression of il-11 in the intact tadpole tails induces expression of the markers for undifferentiated cells. Our results strongly suggest that IL-11 plays a key role in the induction and maintenance of undifferentiated progenitor cells across cell lineages during Xenopus tadpole tail regeneration. il-11 is induced after tail amputation First, we examined the correlation between the cellular processes and il-11 expression in regenerating Xenopus tadpole tails. Quantitative reverse transcription-polymerase chain reaction (qRT-PCR) of il-11 mRNA in the amputated tail stumps of tadpoles collected at 0, 0.5, 1, 2 and 5 h post amputation (hpa) showed that the il-11 expression began at 2 hpa (Fig. 1a ), suggesting that il-11 is related to early events immediately after tail amputation. We then examined il-11 expression levels in later phases after amputation (24, 72 and 120 hpa). il-11 expression was maintained for at least 120 hpa (Fig. 1b ), suggesting that il-11 is also related to some late events after tail amputation. Fig. 1 il-11 is expressed at the tip of blastema during tail regeneration. a , b Expression levels of il-11 were measured by qRT-PCR using RNA extracted from ~20 tadpoles. Tail stump tissues cut at the level of 0.5 mm anterior from the amputated plane were used. Vertical axes represent relative expression levels of il-11 normalised by those of ef1α . Mean ± s.e.m. n = 4. ND: not detected. c – f WISH was performed using tadpoles fixed at 0 c , 24 d , 72 e , or 120 hpa f . Anterior is to the left and dorsal is up . Blue / purple colour represents signals for il-11 expression. Brown pigments are melanophores of the tadpoles. Scale bars : 500 μm. Numbers at the bottom corner indicate the total ratio of tadpoles showing the corresponding expression pattern from at least two batches. Note that il-11 was expressed at the blastema tip at 72 and 120 hpa ( black arrowheads ) Full size image Whole-mount in situ hybridisation (WISH; Fig. 1c–f , Supplementary Fig. 1 ) revealed no significant il-11 expression at 0 hpa at the amputated tail stumps, coinciding with the qRT-PCR results. Significant il-11 expression was detected at the outer edge of the notochord and spinal cord near the amputation plane at 5 and 24 hpa, indicating that il-11 expression was restricted to the amputation plane at the early phase of tail regeneration. At 72 and 120 hpa, il-11 expression was detected at the tip of the regenerating tails, where the tail blastema cells are located (Fig. 1e, f ). We previously observed that proliferating tail blastema cells begin to accumulate at the tip of the regenerating tails 3 days post amputation (dpa) [4] . Induction of il-11 expression at the amputated tail stumps in the early phases (5 and 24 hpa) and its suspension at the tip of regenerating tails in the later phases (>3 dpa) led us to hypothesise that il-11 is involved in the induction and/or maintenance of tail blastema cells, which are undifferentiated progenitor cells of various tissues in the tail. To investigate whether il-11 is selectively expressed among IL-6 family members, we performed qRT-PCR for il-6 and lif , which encode IL-6 family members important for the differentiation or maintenance of stem/progenitor cells [14] , [15] , [16] . Expression of these two genes was modestly induced (at most, less than approximately threefold) after tail amputation compared to the expression of il-11 (Supplementary Fig. 2a–d ), suggesting that il-11 has a specific function in tail regeneration among IL-6 family members. To investigate whether IL-11 signalling is actually activated, we visualised activation of Stat3, which is the major signalling molecule and transcription factor downstream of IL-11 [10] , [11] , by immunohistochemistry using an antibody against phosphorylated Stat3. We found that phosphorylated Stat3 co-localised with the nuclei in notochord bud, spinal cord ampulla and epithelium in blastema of 72-hpa tadpoles (Supplementary Fig. 3 ). Although Stat3 is activated by several upstream ligands, including IL-6 and Lif, expression of these two ligands was not prominently elevated compared to that of il-11 after tail amputation, as mentioned above, and thus it is plausible that the observed activation of Stat3 is mainly due to the expression of IL-11, and that IL-11 signalling is activated in various cell types in blastema. To investigate whether IL-11–responsive cells are induced after tail amputation, we performed qRT-PCR for il11ra and il6st , which are genes for receptors of IL-11 [6] , [7] . Expression of these genes was modestly induced (at most, less than approximately threefold; Supplementary Fig. 2e–h ) compared to the expression of il-11 , suggesting that the IL-11–responsive cells constitutively reside in intact tails and the number of the cells remains largely unaltered during the regeneration process. il-11 is necessary for tail regeneration We next examined whether il-11 is necessary for tail regeneration by knocking-down il-11 using the CRISPR/Cas9 system. Because X. laevis has a long generation time of more than 1 year, we attempted to analyse the effect of il-11 KD in F 0 tadpoles. To efficiently knockdown il-11 in F 0 tadpoles, we designed guide RNAs (gRNAs) targeting two regions each in two il-11 homoeologues of allotetraploid X. laevis , il-11.L and il-11.S (Fig. 2a ), which is expected to cause a large deletion of the nucleotide sequences sandwiched by the two gRNA target sites, in addition to the frame shift that occurs at each of the two gRNA target sites of each gene. We co-injected these gRNAs (#1U.LS, #1D.L and #1D.S) and cas9 mRNA into fertilised eggs, and kept the hatched tadpoles till approximately stage 40–42. We then amputated the tails of F 0 tadpoles ( il-11 KD #1 tadpoles) at 6 days post fertilisation (dpf), and measured the regenerated tail length at 7 dpa (13 dpf). To confirm that the observed phenotype was not due to an off-target effect, we also created another group of KD tadpoles ( il-11 KD #2 tadpoles) using another gRNA set targeting other sequences in il-11 (Fig. 2a ), and compared the regenerated tail length of il-11 KD #1, #2 and control cas9 mRNA-injected tadpoles ( cas9 tadpoles). We detected a loss of genomic regions between the two gRNA target sites of il-11.L and il-11.S using PCR amplification of the interval regions (Fig. 2b–e ), indicating that il-11 genes could be edited by this approach. 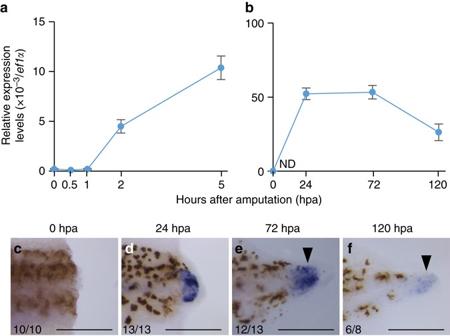Fig. 1 il-11is expressed at the tip of blastema during tail regeneration.a,bExpression levels ofil-11were measured by qRT-PCR using RNA extracted from ~20 tadpoles. Tail stump tissues cut at the level of 0.5 mm anterior from the amputated plane were used.Vertical axesrepresent relative expression levels ofil-11normalised by those ofef1α. Mean ± s.e.m.n= 4. ND: not detected.c–fWISH was performed using tadpoles fixed at 0c, 24d, 72e, or 120 hpaf. Anterior is to theleftand dorsal isup.Blue/purple colourrepresents signals foril-11expression.Brown pigmentsare melanophores of the tadpoles.Scale bars: 500 μm. Numbers at thebottom cornerindicate the total ratio of tadpoles showing the corresponding expression pattern from at least two batches. Note thatil-11was expressed at the blastema tip at 72 and 120 hpa (black arrowheads) The ratio of normally developed il-11 KD tadpoles was not prominently lower than that of cas9 tadpoles (Supplementary Table 1 ), suggesting that il-11 KD does not affect normal development under these conditions. The ratio of normally grown il-11 KD tadpoles after tail amputation was almost the same as that of cas9 tadpoles (Supplementary Table 1 ), suggesting that il-11 does not have a crucial role in wound healing or in immune responses after tail amputation. When we measured relative regenerated tail length normalised by snout to vent length (Supplementary Fig. 4f and g ), we found that the regenerated tail length was significantly shorter in both il-11 KD #1 and #2 tadpoles compared to cas9 tadpoles ( P < 0.05, Dunnett’s test, Fig. 2f–i , Supplementary Fig. 4h ), suggesting that il-11 is necessary for tail regeneration. Deletion of genomic regions between the two gRNA target sites of il-11.L and il-11.S was detected in the tail stump tissues of most of these tadpoles (Supplementary Fig. 4a–e ), suggesting that the function of IL-11 was lost in at least some cells at the amputated tail stumps of most of these il-11 KD tadpoles. Fig. 2 Knockdown of il-11 in tadpoles. a Schematic drawing of genomic structure of il-11 . Bars: introns , orange boxes : untranslated regions, blue boxes : coding sequences, dark grey vertical arrows : gRNA target sequences, light grey horizontal arrows : primers. b – e , Genomic sequences of tadpoles injected with cas9 mRNA and gRNAs. Genomic DNA was extracted from all body of il-11 KD #1 tailbud embryos b , c or tail of il-11 KD #2 tadpoles d , e , and sequences corresponding to il-11.L b , d or il-11.S c , e were PCR-amplified using P1U.L/P1D.L b , P1U.S/P1D.S c , P2U.L/P2D.L d , or P2U.S/P2D.S e primers. The PCR product of the expected length corresponding to deletion of the region between two gRNA target sites was sequenced. Blue characters : reference genomic sequences nearby gRNA target sites, red characters : mismatches from reference genomic sequences, bars : gaps, arrowheads : predicted cleavage sites. Numbers at the left corner indicates ratio of clones containing the sequence to total clones sequenced. f – i , Representative images of tails of control cas9 mRNA-injected f , il-11 KD #1 g , or il-11 KD #2 h tadpoles at 7 dpa, and the tail regeneration length i are shown. Dark-field images f – h are shown. Anterior is to the left , dorsal is up . White broken lines indicate amputated plane. Scale bars : 1 mm. Regeneration length was normalised by snout to vent length (SVL). Box plots are inserted in the panels. Bars in the boxes represent median, upper and lower limits of the boxes represent the first and third quartiles, and whiskers represent maximum and minimum values. * P < 0.05, Dunnett’s test Full size image To confirm that the shortened regeneration length was not due to a non-specific effect of chromosomal disruption, which might have been caused by genome editing, we performed a rescue experiment of the phenotype of il-11 KD tadpoles. For this, an il-11 rescue construct that expresses IL-11 with the expression marker AcGFP upon doxycycline treatment by the tet-on system (Fig. 3a ), or a control construct that expresses AcGFP alone, was co-injected with cas9 mRNA and gRNAs targeting il-11 into a one-cell stage embryo. In the il-11 rescue and control acgfp -expressing constructs, the target sequence of gRNA #1U.LS was inserted. Some constructs might be knocked into the il-11 gene locus by homology-independent double-strand break repair [19] when the genomic il-11 locus and the target sequence on the rescue construct were cleaved concurrently by the CRISPR/Cas9 system (Fig. 3b ). In addition to the free constructs remaining in the cells of the tadpole tail at the time of tail amputation, the knocked-in constructs would facilitate the expression of il-11 by stably inserting into the genome. The injected tadpoles were kept till approximately stage 40–41, then their tails were amputated at 6 dpf following doxycycline treatment, and their regenerated tail length was measured at 7 dpa (13 dpf; Fig. 3c , Supplementary Fig. 5a , b). 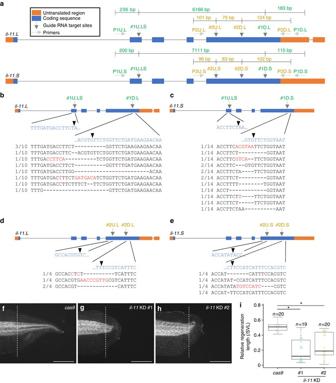Fig. 2 Knockdown ofil-11in tadpoles.aSchematic drawing of genomic structure ofil-11. Bars:introns,orange boxes: untranslated regions,blue boxes: coding sequences,dark greyvertical arrows: gRNA target sequences,light grey horizontal arrows: primers.b–e, Genomic sequences of tadpoles injected withcas9mRNA and gRNAs. Genomic DNA was extracted from all body ofil-11KD #1 tailbud embryosb,cor tail ofil-11KD #2 tadpolesd,e, and sequences corresponding toil-11.Lb,doril-11.Sc,ewere PCR-amplified using P1U.L/P1D.Lb, P1U.S/P1D.Sc, P2U.L/P2D.Ld, or P2U.S/P2D.Seprimers. The PCR product of the expected length corresponding to deletion of the region between two gRNA target sites was sequenced.Blue characters: reference genomic sequences nearby gRNA target sites,red characters: mismatches from reference genomic sequences,bars: gaps,arrowheads: predicted cleavage sites. Numbers at theleft cornerindicates ratio of clones containing the sequence to total clones sequenced.f–i, Representative images of tails of controlcas9mRNA-injectedf,il-11KD #1g, oril-11KD #2htadpoles at 7 dpa, and the tail regeneration lengthiare shown. Dark-field imagesf–hare shown. Anterior is to theleft, dorsal isup.White broken linesindicate amputated plane.Scale bars: 1 mm. Regeneration length was normalised by snout to vent length (SVL).Box plotsare inserted in the panels.Barsin the boxes represent median, upper and lower limits of the boxes represent the first and third quartiles, and whiskers represent maximum and minimum values. *P< 0.05, Dunnett’s test To select tadpoles in which the constructs were successfully introduced, normally grown tadpoles with GFP signal at the amputation plane were selected under a fluorescence stereomicroscope for measurement of the regeneration length of tadpoles with forced acgfp or il-11 expression (Supplementary Table 2 ). In the cas9 group, all normally grown tadpoles were selected, because cas9 tadpoles do not show GFP signals (Supplementary Table 2 ). Although the relative regenerated tail length of il-11 KD acgfp -expressing construct-introduced tadpoles was significantly shorter compared to cas9 mRNA-injected tadpoles, the tail shortening was almost completely rescued in il-11 -rescued tadpoles ( P < 0.05, Tukey−Kramer’s test, Fig. 3d–j , Supplementary Fig. 5c ), suggesting that il-11 is necessary for tail regeneration. Fig. 3 Rescue experiment of the phenotype of il-11 KD tadpoles. a Schematic drawing of a rescue construct. Yellow boxes represent cis-regulatory elements, and green boxes represent coding sequences. gRNA #1U.LS target site was inserted in the construct. In the control construct, acgfp was inserted instead of il-11-p2a peptide-acgfp . b Schematic drawing of knock-in and knockdown. Bars : introns, orange boxes : untranslated regions, blue boxes : coding sequences, dark grey arrows : gRNA target sequences. c Schematic drawing of a rescue experiment. d – j Representative images of tails of control cas9 mRNA-injected d , e , il-11 knockeddown acgfp -expressing f , g , or il-11 knockeddown il-11 –expressing h , i tadpoles, and their regeneration length j are shown. k , Schematic drawing of a rescue experiment using tadpoles treated with or without doxycycline. l-x Representative images of tails of untreated cas9 mRNA-injected l , m , il-11 knockeddown acgfp -expressing n , o , or il-11 knockeddown il-11 –expressing p , q tadpoles, or doxycycline-treated cas9 mRNA-injected r , s , il-11 knockeddown acgfp -expressing t , u , or il-11 knockeddown il-11 –expressing v , w tadpoles and their regeneration length x are shown. Dark-field images d , f , h , l , n , p , r , t , v and GFP2-filtered images e , g , i , m , o , q , s , u , w are shown. Regeneration length was normalised by snout to vent length (SVL). Box plots are inserted in the panels. Bars in the boxes represent median, upper and lower limits of the boxes represent the first and third quartiles, and whiskers represent maximum and minimum values. Scale bars : 1 mm. Anterior is to the left , dorsal is up . Yellow broken lines indicate outline of the tails. White broken lines indicate amputated plane. * P < 0.05, Tukey−Kramer’s test Full size image We also investigated whether the rescue effect is specific for il-11 among the IL-6 family members by forcing the expression of il-6 in il-11 KD tadpoles. 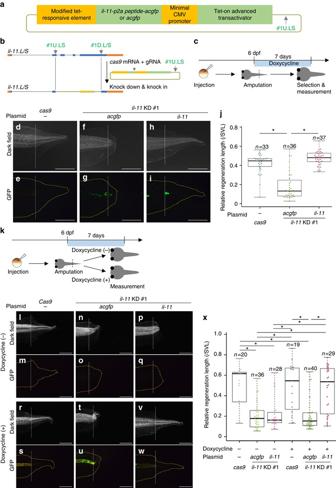Fig. 3 Rescue experiment of the phenotype ofil-11KD tadpoles.aSchematic drawing of a rescue construct.Yellow boxesrepresent cis-regulatory elements, andgreen boxesrepresent coding sequences. gRNA #1U.LS target site was inserted in the construct. In the control construct,acgfpwas inserted instead ofil-11-p2a peptide-acgfp.bSchematic drawing of knock-in and knockdown.Bars: introns,orange boxes: untranslated regions,blue boxes: coding sequences,dark grey arrows: gRNA target sequences.cSchematic drawing of a rescue experiment.d–jRepresentative images of tails of controlcas9mRNA-injectedd,e,il-11knockeddownacgfp-expressingf,g, oril-11knockeddownil-11–expressingh,itadpoles, and their regeneration lengthjare shown.k, Schematic drawing of a rescue experiment using tadpoles treated with or without doxycycline.l-xRepresentative images of tails of untreatedcas9mRNA-injectedl,m,il-11knockeddownacgfp-expressingn,o, oril-11knockeddownil-11–expressingp,qtadpoles, or doxycycline-treatedcas9mRNA-injectedr,s,il-11knockeddownacgfp-expressingt,u, oril-11knockeddownil-11–expressingv,wtadpoles and their regeneration lengthxare shown. Dark-field imagesd,f,h,l,n,p,r,t,vand GFP2-filtered imagese,g,i,m,o,q,s,u,ware shown. Regeneration length was normalised by snout to vent length (SVL).Box plotsare inserted in the panels.Barsin the boxes represent median, upper and lower limits of the boxes represent the first and third quartiles, andwhiskersrepresent maximum and minimum values.Scale bars: 1 mm. Anterior is to theleft, dorsal isup.Yellow broken linesindicate outline of the tails.White broken linesindicate amputated plane. *P< 0.05, Tukey−Kramer’s test Normally grown tadpoles with GFP signal at the amputation plane were selected for measurement of the regeneration length (Supplementary Table 3 ). Regeneration length was almost the same in il-11 KD tadpoles with forced expression of il-6 compared to il-11 KD tadpoles expressing acgfp (Fig. 4 ), suggesting that signalling pathways specific to il-11 among IL-6 family members are necessary for tail regeneration. Fig. 4 il-6 does not rescue the shortened regeneration length of il-11 KD tadpoles. a – f Representative images of tails of control cas9 mRNA-injected a , b , il-11 knockeddown acgfp -expressing c , d , or il-11 knockeddown il-6 –expressing e , f tadpoles, and their regeneration length g are shown. Dark-field images a , c , e and GFP2-filtered images b , d , f are shown. Regeneration length was normalised by snout to vent length (SVL). h , i , SVL h and regeneration length i used for calculation in g are shown. j Biological replicates using different batches of tadpoles are shown. Box plots are inserted in the panels. Bars in the boxes represent median, upper and lower limits of the boxes represent the first and third quartiles, and whiskers represent maximum and minimum values. Scale bars : 1 mm. Anterior is to the left , dorsal is up . Yellow broken lines indicate outline of the tails. White broken lines indicate amputated plane. * P < 0.05, Tukey−Kramer’s test Full size image To further confirm that the rescue effect of il-11 is not due to the introduced construct itself, but to the expression of il-11 , we compared the regeneration length of doxycycline-treated and untreated tadpoles. Injected tadpoles were divided into two groups after tail amputation at 6 dpf: the first group was maintained in 0.1× Steinberg’s solution and the second group was maintained in 0.1× Steinberg’s solution with 50 μg/ml of doxycycline, and regeneration length was measured at 7 dpa (Fig. 3k ). 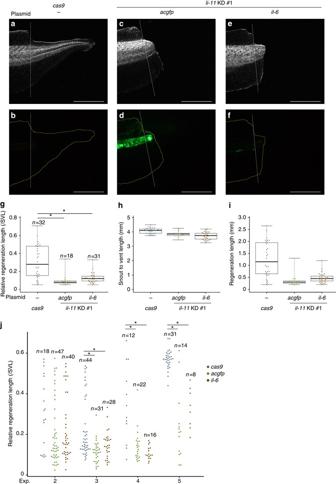Fig. 4 il-6does not rescue the shortened regeneration length ofil-11KD tadpoles.a–fRepresentative images of tails of controlcas9mRNA-injecteda,b,il-11knockeddownacgfp-expressingc,d, oril-11knockeddownil-6–expressinge,ftadpoles, and their regeneration lengthgare shown. Dark-field imagesa,c,eand GFP2-filtered imagesb,d,fare shown. Regeneration length was normalised by snout to vent length (SVL).h,i, SVLhand regeneration lengthiused for calculation ingare shown.jBiological replicates using different batches of tadpoles are shown. Box plots are inserted in the panels.Barsin the boxes represent median, upper and lower limits of the boxes represent the first and third quartiles, andwhiskersrepresent maximum and minimum values.Scale bars: 1 mm. Anterior is to theleft, dorsal isup.Yellow broken linesindicate outline of the tails.White broken linesindicate amputated plane. *P< 0.05, Tukey−Kramer’s test The ratio of normally grown tadpoles after tail amputation was not prominently different between the doxycycline-treated and untreated groups (Supplementary Table 4 ), suggesting that doxycycline treatment did not affect tadpole viability under these conditions. The regeneration length of all normally developed tadpoles was measured and normalised by the snout to vent length (Supplementary Fig. 5d, e ). GFP signals were very weak in untreated acgfp- and il-11 −expressing construct-introduced tadpoles compared to their doxycycline-treated counterparts (Fig. 3o, q, u, w ), suggesting that the expression of AcGFP and IL-11 is doxycycline-dependent. In the untreated group, regeneration length was significantly shorter both in acgfp- and il-11 −expressing construct-introduced tadpoles compared to cas9 tadpoles (Fig. 3l–q, x , Supplementary Fig. 5f ). In the doxycycline-treated group, however, regeneration length was significantly shorter in acgfp -expressing construct-introduced tadpoles compared to il-11 −expressing construct-introduced and cas9 tadpoles, and the regeneration length of il-11 –expressing construct-introduced tadpoles was almost the same as that of cas9 tadpoles ( P < 0.05, Tukey−Kramer’s test, Fig. 3r–w, x , Supplementary Fig. 5f ), clearly indicating that il-11 is necessary for tail regeneration. il-11 induces and maintains progenitors of several tissues Next, to analyse the role of il-11 in tail regeneration, we compared gene expression profiles between the amputated tail stumps of il-11 KD and cas9 tadpoles. When we compared the morphology of regenerating tails of il-11 KD and cas9 tadpoles every day after tail amputation, they were almost the same until 2 dpa. At 3 dpa, however, cas9 tadpoles showed prominent growth of the regenerated tail, whereas il-11 KD tadpoles showed only moderate growth (Supplementary Fig. 6 ), suggesting that some regenerative processes present between 2 and 3 dpa were disrupted in il-11 KD tadpoles. Therefore, we compared gene expression profiles in tail stump tissues of il-11 KD #1 and cas9 tadpoles at 2 dpa by RNA-sequencing. We found that among top 10 genes which showed highest upregulation in il-11 KD #1 tadpoles, five genes are reported to be selectively expressed in skeletal muscle in mouse (Fig. 5a and Supplementary Fig. 7 ), suggesting that ratio of mature tissues were relatively high in tail stump tissues of il-11 KD tadpoles compared to cas9 tadpoles. This prompted us to hypothesise that ratio of undifferentiated cells were relatively high in tail stump tissues of cas9 tadpoles compared to il-11 KD tadpoles. Then we found that the expression levels of several undifferentiated cell markers were affected by il-11 knockdown (Fig. 5a, b ). In il-11 KD #1 tadpoles compared to cas9 tadpoles, we observed a tendency toward or significant (adjusted P < 0.05, Wald test) downregulation of notochord homeobox ( not ), an early notochord marker in Xenopus [20] , [21] ; doublecortin ( dcx ), a marker for a subpopulation of muscle progenitor cells in mouse [22] , [23] ; and runt related transcription factor 1 ( runx1 ), a marker of progenitor cells of Rohon-Beard sensory neurons [24] , which are a subpopulation of primary sensory neurons located in the dorsal spinal cord that mediate the response to touch in larval stages of lower vertebrates. Fig. 5 il-11 induces or maintains tissue progenitor cells across cell lineages during tail regeneration. a Gene expression profile of il-11 KD #1 and cas9 tadpoles. Left panel : volcano plot. Fold-change of expression level of il-11 KD #1 tadpoles over control tadpoles measured by RNA-sequencing are plotted on horizontal axis in log 2 scale, and adjusted P -values are plotted on vertical axis in –log 10 scale. Genes with significant fold-changes (adjusted P < 0.05) are plotted in red . Points beyond the range are plotted on the edge of the graph. Representative undifferentiated markers are plotted in blue . Right panel : top 10 genes which showed highest upregulation in il-11 KD #1 are listed. Mouse homologues of genes indicated in orange are reported to be selectively expressed in skeletal muscle in mice (Supplementary Fig. 7 ). These genes correspond to orange plots in the left panel . b Fold-change of expression levels of representative undifferentiated markers measured by RNA-sequencing. Mean ± s.e.m. n = 3. *adjusted P < 0.05, Wald test. c – h , Localisation of undifferentiated markers. Representative WISH images for not c , f , dcx d , g , or runx1 e , h in control c – e or il-11 KD #1 tadpoles f – h are shown. Anterior is to the left , dorsal is up . Blue / purple colour represents signals for the genes. Brown pigments are melanophores of the tadpoles. Scale bars : 500 μm. Numbers at the bottom corner indicate the total ratio of tadpoles showing the corresponding expression pattern from two batches Full size image When we performed WISH (Fig. 5c–h , Supplementary Fig. 8 ), not was expressed at the tip of the notochord bud, dcx was expressed in the muscle near the amputation plane, and runx1 was expressed in the spinal cord ampulla and ventral side of the blastema. The ratio of tadpoles with strong expression of the genes tended to be higher in the cas9 group ( not : 10/10, dcx : 10/10, and runx1 : 9/10) compared to the il-11 KD #1 and #2 groups ( not : 4/10 and 1/10; dcx : 3/10 and 3/10; runx1 : 6/10 and 7/10). These results suggest that induction and/or maintenance of the progenitor cells of the notochord, muscle, or Rohon-Beard sensory neurons are impaired in il-11 KD tadpoles. We also performed section ISH for the undifferentiated marker genes using doxycycline-treated cas9 mRNA-injected, acgfp- or il-11 −expressing il-11 KD tadpoles fixed at 2 dpa. We detected signals for not and dcx . Expression of not was detected in the notochord bud, and expression of dcx was detected in the muscle and spinal cord (Supplementary Fig. 9 ). The ratio of tadpoles with strong expression in the notochord bud ( not ) or muscle ( dcx ) tended to be higher in cas9 ( not : 6/6, dcx : 11/11) and il-11 -rescued ( not : 6/6. dcx : 11/11) tadpoles compared to control acgfp- expressing il-11 KD tadpoles ( not : 2/6, dcx : 3/11), further suggesting that induction and maintenance of undifferentiated cells are il-11– dependent. The expression of dcx in the spinal cord seems to be il-11 independent, because signals for dcx in the spinal cord were observed in tadpoles in all groups. il-11 can induce progenitor cells in intact tail Finally we examined whether expression of il-11 is sufficient for the induction and/or maintenance of the progenitor cells even in intact tails. For this, we co-injected acgfp - or il-11 –expressing vector with cas9 mRNA and gRNA targeting the tyrosinase locus, which is the gene responsible for albinism and unnecessary for tadpole survival, into the one-cell stage embryo to facilitate the expression of il-11 by construct knocked into the tyr locus, as well as free plasmid retained in the cells of the tadpole tails. Then, the injected tadpoles at 5 dpf (approximately stage 40–42) were treated with doxycycline for 2 days, and the expression levels of the undifferentiated cell marker genes in their tails were compared (Fig. 6a–g ). Although not expression was scarcely detected, or detected at very low levels in acgfp -expressing tails, it was detected in il-11 –expressing tails (Fig. 6h , Supplementary Fig. 10a ). dcx was significantly upregulated in il-11 –expressing tails compared to acgfp -expressing tails ( P < 0.05, Student’s t -test, Fig. 6i , Supplementary Fig. 10b ). The expression level of runx1 tended to be higher in il-11 –expressing tails than in acgfp -expressing tails (Fig. 6j , Supplementary Fig. 10c ). Fig. 6 il-11 is sufficient for induction of progenitor cells across cell lineages in intact tadpole tail. a Schematic drawing of a construct for forced expression of il-11 . Yellow boxes represent cis-regulatory elements, and green boxes represent coding sequences. gRNA #tyr target site was inserted in the construct. In the control construct, acgfp was inserted instead of il-11-p2a peptide-acgfp . b Schematic drawing of knock-in. Dark grey arrows : gRNA #tyr target sequences. c Schematic drawing of a gain of function experiment. d – g , Representative images of tadpoles used in this experiment. acgfp - d , e or il-11 - f , g expressing tails 2 days after doxycycline treatment are shown. Tail tissues indicated in white broken lines from approximately 10 tadpoles were used for qRT-PCR. Dark-field images d , f and GFP2-filtered images e , g are shown. Scale bars : 1 mm. Anterior is to the left , dorsal is up . Yellow broken lines indicate outline of the tails. h – j , Expression levels of not h , dcx i , or runx1 j in tails expressing acgfp or il-11 were measured by qRT-PCR. Vertical axes represent relative expression levels normalised by those of ef1α . Mean ± s.e.m. n = 3. k , l , n , o , Representative ISH images for not k , l or dcx n , o in acgfp k , n or il-11 l , o -expressing intact tadpole tails 2 days after doxycycline treatment are shown. Several not -expressing cells in the notochord sheath ( blue arrowheads ) and dcx -expressing muscle ( red arrowheads ) were detected in il-11 −expressing tails. m The number of not -expressing cells in the notochord sheath in all sections containing notochord was counted. p The ratio of sections containing dcx -expressing muscle in all sections containing muscle was calculated. Box plots are inserted in the panels. Bars in the boxes represent median, upper and lower limits of the boxes represent the first and third quartiles, and whiskers represent maximum and minimum values. Scale bars : 100 μm except inset in (l) (10 μm). Anterior is to the left , dorsal is up . Magenta / purple colour represents signals for the genes. Inset : magnified view of boxed area. * P < 0.05, Student’s t -test. ND: not detected Full size image To investigate whether the number of cells expressing undifferentiated marker genes is increased by forced expression of il-11 , we performed section ISH. We detected signals for not and dcx . not signals were detected in cells in the notochord sheath of il-11 –expressing tadpoles, whereas few signals were detected in acgfp -expressing cells (Fig. 6k–m , Supplementary Fig. 11a ). dcx signals were detected in the spinal cord and muscle (Fig. 6n, o , Supplementary Fig. 11b ). The ratio of muscle expressing dcx was higher in il-11 –expressing tadpoles compared to acgfp -expressing tadpoles (Fig. 6p ), suggesting that IL-11 is sufficient to induce and maintain progenitor cells even in intact tails. Notably, the fact that the genes upregulated in il-11 –expressing tails were undifferentiated cell markers of different tissues suggests that induction of IL-11 alone is sufficient to induce progenitor cells derived from multiple tissues in intact tail, without additional factors that are induced by tail amputation. In the present study, we first analysed the expression of il-11 . il-11 was expressed in the spinal cord and notochord at the amputation plane early after tail amputation, and continued to be expressed in the tip of the spinal cord ampulla and notochord bud in later phases of regeneration (Supplementary Fig. 1g, h ). These regions correspond to the area where runx1- or not- expressing cells reside (Supplementary Figs. 8k, m, o, q , 9a–c ). Therefore, il-11 might induce and maintain these progenitor cells in an autocrine/paracrine manner. Next, we investigated whether il-11 is necessary for tail regeneration by creating il-11 KD/rescue tadpoles. In il-11 -rescued tadpoles, GFP signals were sparse (Fig. 3i, w ). It is important to note that IL-11 is cleaved from AcGFP at the P2A peptide, and therefore GFP signals reflect the localisation of not IL-11 itself, but of il-11 −expressing cells. One possible explanation for how the sparse expression of il-11 could rescue the shortened regeneration length is that IL-11 was very strongly expressed in the source cells and secreted everywhere in the tail at a high concentration, and IL-11–responsive cells that express IL-11 receptors at the tip of the blastema received the IL-11 signal. The result that the forced expression of il-11 in the intact tail prominently upregulated expression of undifferentiated marker genes (Fig. 6 ) supports the idea that the concentration of IL-11 is sufficient for undifferentiated cells to respond even though the GFP signal was sparse. Because we did not observe additional tails or mass in the tails with forced il-11 expression, it is possible that additional signals at the tip of the blastema are needed for prolonged survival or continued proliferation of the progenitor cells. We then analysed the role of il-11 in tail regeneration. We found that marker genes of progenitor cells in different cell lineages were downregulated in il-11 KD tadpoles (Fig. 5 ), and upregulated in tadpoles with forced il-11 expression (Fig. 6 ). Notably, these marker genes were not exclusively expressed in a single cell population. dcx was expressed in the spinal cord (Fig. 6n, o , Supplementary Figs. 8 l, n, p, 9 e–h, 11b ) as well as in muscle. dcx is expressed in neuronal precursor cells in the developing mouse brain [25] . Therefore, it is possible that these cells are neural progenitors, although they might be il-11 independent, because the signal for dcx in the spinal cord was not prominently downregulated in il-11 KD tadpoles (Supplementary Figs. 8 n, p, 9h ), or upregulated in tadpoles with forced expression of il-11 (Fig. 6n, o , Supplementary Fig. 11b ). runx1 was expressed in the ventral region of the amputated tail stumps in addition to the spinal cord (Supplementary Fig. 8m, o, q ). runx1 is expressed in hemogenic endothelium in mice [26] . The dorsal aorta is located at the ventral side of the Xenopus tadpole tail. Therefore, runx1 might also be expressed in the postulated hemogenic endothelium at the amputated plane in Xenopus . Further studies, such as lineage tracing of cells expressing the markers or transplantation analysis of the progenitors will more strongly support the idea that the cells induced and maintained by il-11 are actually progenitor cells of various cell lineages. Although previous studies reported that il-11 is expressed in regenerating heart in zebrafish [18] , and that IL-11 maintains expression of undifferentiated markers in human embryonic stem cells [17] , our findings are the first to indicate that IL-11 plays a key role in the induction and maintenance of the progenitor cells of various tail tissues. Downstream of IL-11, it is probable that some intracellular signals, which have been investigated in mammals [5] , function to maintain a broad range of stem/progenitor cells in an undifferentiated state. Analysing the molecular mechanisms that link tail amputation to il-11 induction, such as the identification of a regeneration-specific enhancer element, which is suggested in zebrafish [27] , will unveil regeneration-specific molecular and cellular processes that start after amputation in organ regeneration. Statistical tests were not used to pre-determine sample size. The experiments were not randomised or blinded. Normally developed tadpoles were used in the experiments. Animals and tail amputation Animals were obtained and treated as described previously [4] . In brief, tadpoles were obtained by mating wild-type Xenopus laevis , and maintained in 0.2% salt water at 20 °C until they were used. Tadpole tails were amputated at 5 days post fertilisation (dpf) (Nieuwkoop and Faber stage [28] 39–42) after anaesthetisation with 0.02% MS-222 (Sigma-Aldrich, St. Louis, MO). We followed the Guidelines for Proper Conduct of Animal Experiments of Science Council of Japan. The protocol in this study was approved by the Committee on the Ethics of Animal Experiments of the Graduate School of Science at the University of Tokyo. qRT-PCR qRT-PCR was performed essentially as described previously [4] with minor modifications. In brief, total RNA was extracted using RNeasy mini kit (Qiagen, Germany), and reverse transcribed using PrimeScript RT reagent Kit with gDNA Eraser (Perfect Real Time; TaKaRa, Japan). Targets were amplified using SYBR premix ExTaq II (Tli RNaseH plus; TaKaRa) and a LightCycler 480 Real-time PCR System (Roche Diagnostics, Switzerland). The amounts of the transcripts were normalised with those of elongation factor-1 alpha ( ef1a) . The forward and reverse primers used for amplification of each gene were as follows: ef1α ; 5′-GGAACGGTGACAACATGC-3′ and 5′-AGGCAGACGGAGAGGCTTA-3′, il-11 ; 5′-TCCTGAAGCTAAGCACTGACCT-3′ and 5′-TGAATTCCGTTAAATTCGTGGTCCA-3′, il-6 ; 5′-TTGTGGCCACTCACCTTGGT-3′ and 5′-GATGAGCTTCGCTAGGGCCA-3′, lif ; 5′-AACAGCGATGCCATTGGACA-3′ and 5′-TGCTCCAGATGCCAGCTCTT-3′, il11ra ; 5′-AATCACATCGCTGGCGTGTG-3′ and 5′-CATCCAGCAGCCGGAAACTG-3′, il6st ; 5′-CCAGAAGCTCCACCTTCCAG-3′ and 5′-CCATTGGCTACGGAGTCACTT-3′, not ; 5′-GAACAGACAGACCTGCCTCC-3′ and 5′-AGCGGTAGGGCATAGATGGG-3′, dcx ; 5′-TGCCGATTCAGCCAATGGAA-3′ and 5′-TGCTTACGAAGGCTTCCTGG-3′, runx1 ; 5′-CAGCCCGCATCACCCAAATC-3′ and 5′-TCTGACCCTGAGGCTGAGGA-3′. WISH WISH was performed as described previously [4] . In brief, whole body of the tadpoles were fixed with MEMFA (50 mM 3-(N-morpholino) propanesulfonic acid, pH 7.4, including 2 mM ethylene glycol-bis(2-aminoethylether)-N,N,N′,N′-tetraacetic acid, 1 mM MgSO 4 , 3.7% formaldehyde) fixative, and kept in methanol at −20 °C until they were stained. Then they were rehydrated, treated with 50 μg/ml of proteinase K for 10 min, treated with 0.5% of acetate anhydride in 0.1 M of triethanolamine, and fixed with 3.7% formaldehyde. The specimens were pre-hybridised in the hybridisation buffer (Denhardt’s solution (Wako, Japan) including 50% formamide, 0.75 M NaCl, 0.075 M trisodium citrate, 100 μg/ml heparin, 0.1% Tween 20, 0.1% 3-((3-Cholamidopropyl) dimethylammonio) propanesulfonate, and 1 mg/ml Ribonucleic acid from torula yeast Type VI (Sigma-Aldrich)) for 4–6 h at 60 °C, and hybridised with the probe solution (1 μg/ml of digoxigenin labelled RNA probe in hybridisation buffer) for 4 nights at 60 °C. They were treated with RNase solution (1% RNase Cocktail (Invitrogen, Waltham, MA) in 0.3 M NaCl and 0.03 M trisodium citrate), following incubation with alkaline phosphatase conjugated anti-digoxigenin antibody and chromogenic reaction with a nitro blue tetrazolium chloride/5-bromo-4-chloro-3-indolyl phosphate, toluidine salt solution. After staining, they were treated with 10% H 2 O 2 in phosphate-buffered saline to bleach the melanophore of the tadpoles, although some of the melanophores remained in the specimens. Following staining, some of the specimens were embedded in 4% agar in phosphate-buffered saline, and sagittally sliced at 30-μm intervals using a vibratome VT1000S (Leica Biosystems, Germany). Immunohistochemistry Immunohistochemistry was performed essentially as described previously [29] . In brief, tadpole tails were amputated at 5 dpf (stage 39–41) and fixed at 3 dpa (stage 47) with MEMFA fixative, embedded with 25% gelatin 15% sucrose, frozen, sagittally sliced at 10 μm thick, and incubated with anti-phospho-Stat3 (Tyr705) mouse antibody (Cell Signalling Technology, MA, #9138S) following incubation with Alexa Fluor 555-conjugated anti-mouse IgG goat antibody (Invitrogen, A-21424). Nuclei were counterstained with 10 μg/ml of Hoechst 33342 (Lonza, Switzerland). Knockdown experiment gRNAs [30] and cas9 [31] mRNA were designed and synthesised essentially as described previously with minor modifications. In brief, DR274 [30] plasmid was digested with Bsa I-HF (New England Biolabs, MA), annealed with oligonucleotide, and they were ligated. Some of the gRNA template plasmids were assembled using a PCR-amplified DR274 fragment, an oligonucleotide, and an In-Fusion HD Cloning Kit (TaKaRa). After transformation and plasmid extraction, the plasmid was digested with Dra I ( Aha III; TaKaRa), following PCR amplification and in vitro transcription using AmpliScribe T7- Flash Transcription Kit (Epicentre, WI). The gRNA was purified using RNeasy mini kit. The number of possible off-target sites of the obtained gRNAs was predicted by searching Xenopus laevis genome 9.1 (Xenbase [32] , [33] ) using Cas-OFFinder [34] and possible gRNAs that recognised any sites other than the target genes in the genome were not used. gRNA target sequences were as follows: #1U.LS; GGTGCATAGCCATGTTTAGAAGG, #1D.L; GGACTATGCAACACGTGTTCTGG, #1D.S; GGACTTTGCAACACGTGTTCTGG, #2U.L; GCACCATATGCCACGTGTCACGG, #2U.S; GTTCCGTGACACGTGGTATATGG, #2D.L; GAGGTGGAAATGACGGAAAATGG, #2D.S; GACGTGGAAATGATGGAAGATGG. For cas9 mRNA synthesis, pXT7-hcas9 [31] (China Zebrafish Resource Center, China, CZP2) was digested with Xba I (TaKaRa), following in vitro transcription using mMESSAGE mMACHINE T7 ULTRA Kit (Invitrogen). The obtained cas9 mRNA was purified using RNeasy mini kit. 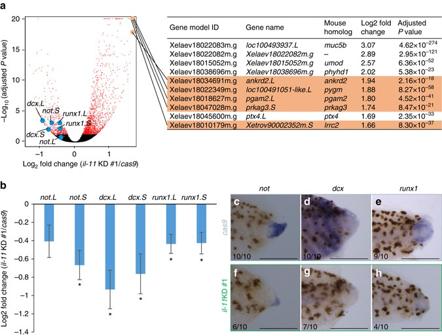Fig. 5 il-11induces or maintains tissue progenitor cells across cell lineages during tail regeneration.aGene expression profile ofil-11KD #1 andcas9tadpoles.Left panel: volcano plot. Fold-change of expression level ofil-11KD #1 tadpoles over control tadpoles measured by RNA-sequencing are plotted on horizontal axis in log2scale, and adjustedP-values are plotted on vertical axis in –log10scale. Genes with significant fold-changes (adjustedP< 0.05) are plotted inred. Points beyond the range are plotted on the edge of the graph. Representative undifferentiated markers are plotted inblue.Right panel: top 10 genes which showed highest upregulation inil-11KD #1 are listed. Mouse homologues of genes indicated inorangeare reported to be selectively expressed in skeletal muscle in mice (Supplementary Fig.7). These genes correspond toorangeplots in theleft panel.bFold-change of expression levels of representative undifferentiated markers measured by RNA-sequencing. Mean ± s.e.m.n= 3. *adjustedP< 0.05, Wald test.c–h, Localisation of undifferentiated markers. Representative WISH images fornotc,f,dcxd,g, orrunx1e,hin controlc–eoril-11KD #1 tadpolesf–hare shown. Anterior is to theleft, dorsal isup.Blue/purple colourrepresents signals for the genes.Brown pigmentsare melanophores of the tadpoles.Scale bars: 500 μm. Numbers at the bottom corner indicate the total ratio of tadpoles showing the corresponding expression pattern from two batches 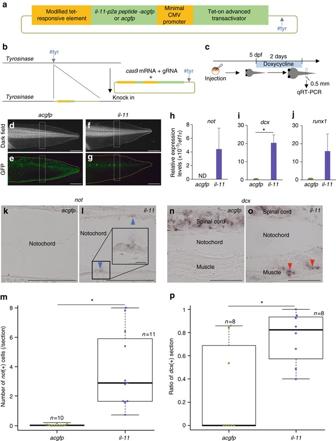Fig. 6 il-11is sufficient for induction of progenitor cells across cell lineages in intact tadpole tail.aSchematic drawing of a construct for forced expression ofil-11.Yellow boxesrepresent cis-regulatory elements, andgreen boxesrepresent coding sequences. gRNA #tyr target site was inserted in the construct. In the control construct,acgfpwas inserted instead ofil-11-p2a peptide-acgfp.bSchematic drawing of knock-in.Dark grey arrows: gRNA #tyr target sequences.cSchematic drawing of a gain of function experiment.d–g, Representative images of tadpoles used in this experiment.acgfp-d,eoril-11-f,gexpressing tails 2 days after doxycycline treatment are shown. Tail tissues indicated inwhite broken linesfrom approximately 10 tadpoles were used for qRT-PCR. Dark-field imagesd,fand GFP2-filtered imagese,gare shown.Scale bars: 1 mm. Anterior is to theleft, dorsal isup.Yellow broken linesindicate outline of the tails.h–j, Expression levels ofnoth,dcxi, orrunx1jin tails expressingacgfporil-11were measured by qRT-PCR.Vertical axesrepresent relative expression levels normalised by those ofef1α. Mean ± s.e.m.n= 3.k,l,n,o, Representative ISH images fornotk,lordcxn,oinacgfpk,noril-11l,o-expressing intact tadpole tails 2 days after doxycycline treatment are shown. Severalnot-expressing cells in the notochord sheath (blue arrowheads) anddcx-expressing muscle (red arrowheads) were detected inil-11−expressing tails.mThe number ofnot-expressing cells in the notochord sheath in all sections containing notochord was counted.pThe ratio of sections containingdcx-expressing muscle in all sections containing muscle was calculated. Box plots are inserted in the panels.Barsin the boxes represent median, upper and lower limits of the boxes represent the first and third quartiles, andwhiskersrepresent maximum and minimum values.Scale bars: 100 μm except inset in (l) (10 μm). Anterior is to theleft, dorsal isup.Magenta/purplecolour represents signals for the genes.Inset: magnified view of boxed area. *P< 0.05, Student’st-test. ND: not detected The injections were carried out essentially as described previously [29] with the modifications. In brief, fertilised eggs obtained by artificial fertilisation were dejellied by incubation with 3% cysteine, following injection in Ficoll solution (2% Ficoll 400 in 10 mM NaCl, 0.2 mM KCl, 0.1 mM MgCl 2 , 0.2 mM CaCl 2 , 0.5 mM 2-(4-(2-Hydroxyethyl)-1-piperazinyl)ethanesulfonic acid, pH 7.5) using Nanoject II (Drummond Scientific Company, PA). We injected cas9 mRNA (700 ng/μl) and gRNAs (20 ng/μl each, #1U.LS, #1D.L, and #1D.S in il-11 KD #1, and #2U.L, #2U.S, #2D.L, and #2D.S in il-11 KD #2) at a volume of 18.4 nl into single-cell stage embryos. Embryos were injected and kept at 12 °C until gastrulation began, and reared at 20 °C thereafter. The tails were amputated from the tadpoles at 6 dpf, and the tail regeneration length was measured at 7 dpa. Genomic DNA was extracted using DNeasy Blood and Tissue kit (Qiagen) or by boiling tissues in 50 mM NaOH at 98 °C for 10 min followed by adding 1/10 volume of 1 M Tris-HCl (pH 7.5). Primers used for amplification of genomic regions around the gRNA target sites and annealing temperatures were as follows: P1U.L and P1D.L; 5′-TGACTCAGTACTGCGATATTTCCA-3′ and 5′-AGGTCCTAAAATGTCCCGGT-3′ (53 °C), P1U.S and P1D.S; 5′-TTTTGCTGGGACTTCGTTGC-3′ and 5′- ACCTCAGGCGTTTGATGCTA-3′ (58 °C), P2U.L and P2D.L; 5′-AGAGTTTCTGGATAATGGACCCC-3′ and 5′-ATATGTGCCCGTTCTGCAGT-3′ (60 °C), P2U.S and P2D.S; 5′-GGAGAGATAACTAAAAGCTAACACAA-3′ and 5′-ACATCAAGGATGGAGGTTTGTGA-3′ (60 °C). Primers used for amplification of positive control ef1α were the same as described in the qRT-PCR section. PCR products were cloned into pGEM-T easy vector (Promega, Madison, WI, USA) and sequenced. The statistical significance of the difference in the relative regeneration length normalised by snout to vent length was assessed by Dunnett’s test or Student’s t -test with a cutoff of P < 0.05. Rescue experiment The rescue construct was assembled using the In-Fusion HD Cloning Kit (TaKaRa). In brief, the il-11 fragment was PCR-amplified using the il-11.L sequence (AB933563) [4] cloned into pGEM-T easy vector (Promega). Fragments containing acgfp , or minimal CMV promoter and Tet-On Advanced transactivator were PCR-amplified using pAcGFP1-N1 (TaKaRa), or pTet-On Advanced (TaKaRa) as templates, respectively. Oligonucleotides for Gly-Ser-Gly-P2A peptide [35] and the gRNA #1U.LS target sequence were as follows: 5′-GGAAGCGGAGCTACTAACTTCAGCCTGCTGAAGCAGGCTGGAGACGTGGAGGAGAACCCTGGACCT-3′ and 5′-AGGTCCAGGGTTCTCCTCCACGTCTCCAGCCTGCTTCAGCAGGCTGAAGTTAGTAGCTCCGCTTCC-3′, 5′-CAGCTCGACCAAGCTCCTTCTAAACATGGCTATGCACC-3′ and 5′-AAATCTCGCCAAGCTGGTGCATAGCCATGTTTAGAAGG-3′. These fragments and oligonucleotides were inserted into pTRE-Tight (TaKaRa). To prevent double-strand breaks, synonymous substitutions were introduced at the target sequence for #1U.LS and #1D.L in the il-11.L sequence of the rescue construct by PCR using mutated primers as follows: 5′- TGATGATTTGCTAAACATGGCTATGCAC-3′ and 5′- TTTAGCAAATCATCAAATTCCACTTTT-3′, 5′-TTGTTCTGATGAAGAACAAGTTGGGA-3′ and 5′-TCTTCATCAGAACAAGAACACGTGTT-3′. For construction of the plasmid used for the forced expression of il-6 , the il-11 sequence of the il-11 rescue construct was substituted by the coding sequence of il-6.S cloned into a pGEM-T easy vector using the In-Fusion system. Injection was carried out as described in the knockdown experiment section except that 6 ng/μl of the rescue construct was added to the injection solution. Tails from injected tadpoles were amputated at 6 dpf, tadpoles were treated with 50 μg/ml doxycycline in 0.2% salt water as described previously [29] for 7 days immediately after tail amputation, and tail regeneration length was measured. Only tadpoles showing green fluorescence near the amputation plane or a regenerated tail were used in the acgfp -expressing and il-11 rescue groups. Tadpoles showing extremely high green fluorescence were excluded to prevent possible adverse effects of a high concentration of AcGFP. This criterion was not pre-established. In experiments comparing the regeneration length of the untreated and doxycycline-treated groups, tadpoles were incubated in either 0.1× Steinberg’s solution (0.3 mM 2-(4-(2- hydroxyethyl)-1-piperazinyl)ethanesulfonic acid, pH 7.4, including 5.8 mM NaCl, 67 μM KCl, 34 μM Ca(NO 3 ) 2 , 83 μM MgSO 4 ) or 0.1× Steinberg’s solution with 50 μg/ml of doxycycline after tail amputation, and the regeneration length of all normally grown tadpoles were measured. The statistical significance of the difference in the relative regeneration length normalised by snout to vent length was assessed by Tukey−Kramer’s test with a cutoff of P < 0.05. RNA-sequencing Library construction, sequencing, and mapping were performed essentially as described previously [4] with the minor modifications. In brief, tail stump tissues cut at the level 0.5 mm anterior from the amputated plane were collected at 2 dpa from ~20 cas9 mRNA-injected or il-11 KD #1 tadpoles from 3 different batches. Total RNA was extracted using RNeasy mini kit. cDNA library was produced using TruSeq Stranded Total RNA with Ribo-Zero Gold LT Sample Prep Kit (Illumina, CA). We produced a set of approximately 5 × 10 7 single end reads (66 bp) from each cDNA library using Hiseq 2500 (Illumina). X. laevis genome 9.1 (Xla.v91.repeatMasked.fa; Xenbase [32] , [33] ) was used as a reference for mapping. The number of reads mapped to each gene was counted using HTSeq [36] with a reference gene model (XL_9.1_v1.8.3.2.primaryTranscripts.gff3; Xenbase [32] , [33] ) and compared using DESeq2 [37] . A volcano plot was created using ggplot2 [38] . Gene expression levels of mouse homologues were obtained from BioGPS [39] , [40] , [41] using a microarray data set of a previous study in mouse [42] . Forced expression in intact tail The gRNA #tyr target sequence was as follows: 5′-GGCTCCATGTCTTCCGTCCAAGG-3′. Although an off-target sequence was found in the latest Xenopus laevis genome 9.1, most tadpoles survived after injection. Construction for forced expression of il-11 was carried out as described in the rescue experiment section except that no mutation was introduced in il-11 sequences, and the gRNA #tyr target sequence was introduced instead of #1U.LS using oligonucleotide as follows: 5′-CAGCTCGACCAAGCTGGCTCCATGTCTTCCGTCCAAGG-3′ and 5′-AAATCTCGCCAAGCTCCTTGGACGGAAGACATGGAGCC-3′ Injection and doxycycline treatment were carried out as described in the rescue experiment section except that concentration of gRNA #tyr was 40 ng/μl, and embryos were maintained at 20 °C after they developed to the 16-cell stage. Doxycycline treatment started at 5 dpf, and continued for 2 days following sampling for qRT-PCR or ISH. Tadpoles with GFP signals in the region approximately corresponding to the tail tissues used for qRT-PCR were used for the analyses. Tissue section ISH ISH was performed essentially as described previously [43] . In brief, tadpoles were fixed with Bouin’s fixative, embedded in Paraplast (McCormick Scientific, St. Louis, MO). Eight micrometre-thick sagittal sections was prepared, and rehydrated. The slides were incubated with digoxigenin-labelled probe solution overnight, following incubation with alkaline phosphatase conjugated anti-digoxigenin antibody and chromogenic reaction with a nitro blue tetrazolium chloride/5-bromo-4-chloro-3-indolyl phosphate, toluidine salt solution. For detection of dcx , tadpoles were fixed with MEMFA instead of Bouin’s fixative. Three probes targeting different regions of dcx were mixed and used to increase detection sensitivity. Data availability RNA-sequencing data have been deposited in the DNA DataBank of Japan under accession code PRJDB5211. We used already deposited GSE10246 data set [42] in Gene Expression Omnibus of NCBI for expression analysis in mouse tissues. High resolution supplementary figures are available at doi:10.6084/m9.figshare.5131867. We declare that all data supporting the findings of this study are available within the article and its supplementary information files or from the corresponding author upon reasonable request.